Controlling superconductivity by tunable quantum critical points The heavy fermion compound CeRhIn 5 is a rare example where a quantum critical point, hidden by a dome of superconductivity, has been explicitly revealed and found to have a local nature. The lack of additional examples of local types of quantum critical points associated with superconductivity, however, has made it difficult to unravel the role of quantum fluctuations in forming Cooper pairs. Here, we show the precise control of superconductivity by tunable quantum critical points in CeRhIn 5 . Slight tin-substitution for indium in CeRhIn 5 shifts its antiferromagnetic quantum critical point from 2.3 GPa to 1.3 GPa and induces a residual impurity scattering 300 times larger than that of pure CeRhIn 5 , which should be sufficient to preclude superconductivity. Nevertheless, superconductivity occurs at the quantum critical point of the tin-doped metal. These results underline that fluctuations from the antiferromagnetic quantum criticality promote unconventional superconductivity in CeRhIn 5 . Strange metallic behaviour arises from incoherent electron scattering by critical fluctuations that emerge from a continuous quantum phase transition at absolute zero temperature [1] , [2] . Unconventional superconductivity is a potential ordered quantum state that subsumes entropy generated by the proliferation of fluctuations emanating from the quantum critical point (QCP) [3] , [4] , [5] . In this case, the spectrum of associated quantum fluctuations determines the structure of the superconducting (SC) gap [6] , [7] , [8] , [9] . Although several classes of unconventional superconductors have been discovered in proximity to a T =0 magnetic instability, the role that associated fluctuations play in forming SC Cooper pairs is still debatable. Often a projected QCP is hidden by superconductivity, but CeRhIn 5 is a rare example where the hidden QCP has been revealed by an applied magnetic field, exposing strange metallic behaviour and emphasizing the close interplay between quantum criticality and superconductivity [4] . However, scarcity of additional examples of a revealed QCP that otherwise is hidden under a SC dome raises the questions of whether unconventional superconductivity is indeed a manifestation of an ordered phase arising from quantum fluctuations and whether that superconductivity can be controlled by a tunable QCP. At atmospheric pressure, the heavy fermion metal CeRhIn 5 orders antiferromagnetically below 3.8 K (= T N ), where spins of Ce 4 f electrons are anti-aligned within the Ce-In plane and rotate incommensurately by 106.9° in the adjacent plane along the tetragonal c axis [10] , [11] . Applied pressure P suppresses T N and induces superconductivity that coexists microscopically with magnetic order up to a critical pressure of 1.75 GPa where, in the absence of an applied magnetic field, Néel order abruptly disappears and is replaced by superconductivity. The dome of pressure-dependent superconductivity T c ( P ) is a maximum at 2.3 GPa, the pressure where the antiferromagnetic (AFM) QCP is revealed by an applied magnetic field [4] . T N of CeRhIn 5 also is suppressed gradually with Sn substitution for In and reaches 0 K at a critical concentration x c =0.07, CeRh(In 1− x Sn x ) 5 (refs 12 , 13 ). A gradual enhancement of the electronic Sommerfeld coefficient of specific heat with decreasing temperature and a sub- T linear dependence of the electrical resistivity at x c are consistent with the non-Fermi-liquid behaviours that are observed at the pressure- and field-induced QCP of pure CeRhIn 5 , but with less singularity possibly due to effects of disorder from Sn substitution that also prevent the development of superconductivity at x c . The variation of T N with Sn concentration suggests that the position of a pressure-induced QCP in a sample with x < x c may be shifted to a lower pressure relative to pristine CeRhIn 5 because Sn doping enhances hybridization between the local Ce 4 f spin and itinerant electrons (as shown in Supplementary Fig. 1 and Supplementary Note 1 ), therefore acting as effective positive pressure. If the unconventional superconductivity of CeRhIn 5 was to arise from an attractive pair interaction mediated by quantum critical fluctuations, pressure-induced superconductivity in lightly Sn-doped CeRhIn 5 would be expected to be controlled by its QCP. In the following, we present electrical resistivity measurements of 4.4% Sn-doped CeRhIn 5 under pressure and magnetic field, which reveals that Sn doping shifts the AFM QCP from 2.3 GPa to 1.3 GPa in undoped CeRhIn 5 . This slight Sn substitution leads to a residual impurity scattering that is 300 times larger at atmospheric pressure than that of pure CeRhIn 5 , which should preclude the possibility of superconductivity. In spite of this strong scattering, pressure-induced superconductivity in the Sn-doped metal emerges and reaches a maximum T c at the QCP of 1.3 GPa. Above T c , the temperature exponent of resistivity is sub-linear, manifesting strange metallic behaviour emanating from the absolute zero temperature instability. Taken together with the precise control of superconductivity by doping- and pressure-tuned QCPs, these results show that it is the QCP that controls the appearance of the unconventional SC phase. Electrical resistivity and anomalous electron scattering The colour contour map in Fig. 1a describes the evolution of absolute values of the c axis electrical resistivity ( ρ c ) of 4.4% Sn-doped CeRhIn 5 at 5 Tesla, a field slightly higher than the SC upper critical field over the whole pressure range studied. Strong enhancement of ρ c is centred around 1.3 GPa, showing a funnel-shape topology. Isothermal resistivity at the base temperature of 0.3 K also is enhanced near 1.3 GPa, being a factor of 1.7 times larger than that at 2.46 GPa (see Supplementary Fig. 2 and Supplementary Note 2 ). In the absence of a magnetic field, as shown in Fig. 1b , a pressure-induced SC phase as well as magnetic order appear. In this limit, T N gradually decreases with pressure and disappears when it becomes smaller than T c ; whereas, T c ( P ) is dome shaped with maximal T c at 1.3 GPa (phase transitions in resistivity are shown in Supplementary Fig. 3b for representative pressures). Although the contour of ρ c is influenced by the presence of new broken symmetries at low temperatures, it shows a similar enhancement of ρ c above T c at the optimal pressure ( P c ). Complete suppression of T N near P c provides compelling evidence that the anomalous enhancement of ρ c in the pressure–temperature plane is a consequence of critical fluctuations from an AFM QCP under the SC dome of Sn-doped CeRhIn 5 . 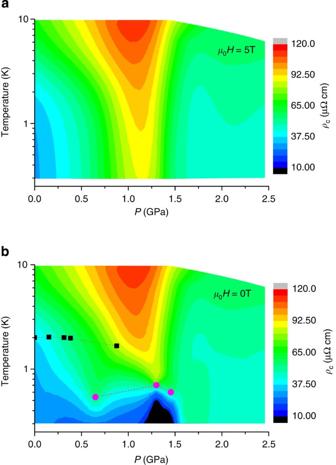Figure 1: Electrical resistivity of 4.4% Sn-doped CeRhIn5under pressure. (a) A contour map of thecaxis electrical resistivity (ρc) is plotted in the pressure–temperature plane for a magnetic field of 5 Tesla, which is slightly larger thanμ0Hc2(0). The colours represent absolute values ofρc, where a funnel of enhanced electronic scattering emerges near 1.3 GPa. (b) Contour map ofρcis plotted for a magnetic field of 0 Tesla. The antiferromagnetic transition and superconducting transition temperatures are plotted in square and circle symbols, respectively.Tcis assigned as the onset point of the phase transition. Data representative of those from which this map was constructed are shown inSupplementary Fig. 3. Figure 1: Electrical resistivity of 4.4% Sn-doped CeRhIn 5 under pressure. ( a ) A contour map of the c axis electrical resistivity ( ρ c ) is plotted in the pressure–temperature plane for a magnetic field of 5 Tesla, which is slightly larger than μ 0 H c2 (0). The colours represent absolute values of ρ c , where a funnel of enhanced electronic scattering emerges near 1.3 GPa. ( b ) Contour map of ρ c is plotted for a magnetic field of 0 Tesla. The antiferromagnetic transition and superconducting transition temperatures are plotted in square and circle symbols, respectively. T c is assigned as the onset point of the phase transition. Data representative of those from which this map was constructed are shown in Supplementary Fig. 3 . Full size image QCP and sub- T linear resistivity The local temperature exponent n of ρ c at 5 Tesla, where n =θlnΔ ρ /θln T and Δ ρ = ρ c − ρ 0 = AT n , also is anomalous near 1.3 GPa, as shown in Fig. 2a . The residual resistivity ρ 0 reflects impurity scattering that depends on both the amount of disorder and the effective impurity potential, which itself is enhanced by critical fluctuations [14] . The colour contour that describes the local exponent n reveals a sub-linear temperature dependence in a narrow pressure–temperature plane around 1.3 GPa and low temperatures, a hallmark of quantum critical behaviour, and the resistivity follows a Fermi-liquid T 2 dependence elsewhere. 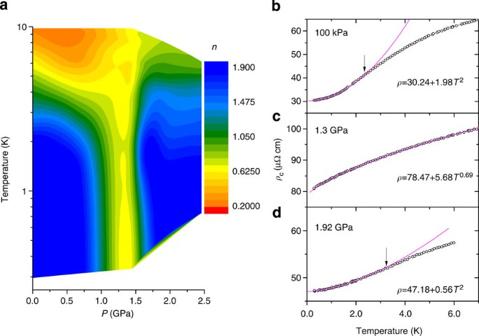Figure 2: Non-Fermi-liquid electrical resistivity (ρc) of 4.4% Sn-doped CeRhIn5under pressure. (a) Colours represent the local exponent,n=θlnΔρ/θlnT, at 5 Tesla, where Δρ=ρc−ρ(T=0 K)=ATn. The resistivityρcwas measured along the crystallinecaxis. The sub-Tlinear dependence ofρcat 1.3 GPa is a hallmark of unconventional non-Fermi liquids. (b) Low temperature resistivityρcis plotted at pressures of 0.001, 1.3 and 1.92 GPa in (b), (c) and (d), respectively. The solid lines are least-squares fits ofρc=ρ(T=0 K)+ATn. The resistivity deviates from Landau–FermiT2behaviour at the QCP (=1.3 GPa), but it follows aT2dependence at pressures away from the QCP. Arrows mark the Fermi liquid temperatureTFLbelow whichρc∝T2and other pressures results are shown inSupplementary Fig. 4. Figure 2b–d representatively show the low temperature ρ c (T) at 5 Tesla for pressures of 100 kPa (< P c ), 1.3 GPa (= P c ) and 1.92 GPa (> P c ) in the top, middle and bottom panels, respectively. At ambient pressure, a Landau–Fermi T 2 dependence is observed below 2.3 K and the residual resistivity is 30.2 μΩ cm, which is about 300 times larger than that of pure CeRhIn 5 (=0.1 μΩ cm) due to potential scattering by impurities. The T 2 coefficient A is 1.98 μΩ cm K −2 , which corresponds to a Sommerfeld-specific heat coefficient γ =445 mJ mol −1 K −2 from the Kadowaki–Woods relation [15] , confirming that Sn-doped CeRhIn 5 is a heavy electron system. At 1.38 GPa, the pressure where T c is a maximum at zero magnetic field, ρ c (T) deviates from a T 2 dependence, following a sub- T linear dependence over an extended temperature range from the base temperature (=0.3 K) to 7 K, that is, ρ c = ρ 0 + AT n with n =0.69 and ρ 0 =78.5 μΩ cm. We note that the fitting parameters are n =0.71 and ρ 0 =5.2 μΩ cm for pure CeRhIn 5 at 2.35 GPa, the QCP, as well as the optimal pressure for superconductivity [16] . Figure 2: Non-Fermi-liquid electrical resistivity ( ρ c ) of 4.4% Sn-doped CeRhIn 5 under pressure. ( a ) Colours represent the local exponent, n =θlnΔ ρ /θln T , at 5 Tesla, where Δ ρ = ρ c − ρ ( T =0 K)= AT n . The resistivity ρ c was measured along the crystalline c axis. The sub- T linear dependence of ρ c at 1.3 GPa is a hallmark of unconventional non-Fermi liquids. ( b ) Low temperature resistivity ρ c is plotted at pressures of 0.001, 1.3 and 1.92 GPa in ( b ), ( c ) and ( d ), respectively. The solid lines are least-squares fits of ρ c = ρ ( T =0 K)+ AT n . The resistivity deviates from Landau–Fermi T 2 behaviour at the QCP (=1.3 GPa), but it follows a T 2 dependence at pressures away from the QCP. Arrows mark the Fermi liquid temperature T FL below which ρ c ∝ T 2 and other pressures results are shown in Supplementary Fig. 4 . Full size image The residual resistivity ρ 0 is much larger in Sn-doped CeRhIn 5 than in pure CeRhIn 5 at their respective critical pressures, but the exponent n at the QCP is independent of disorder, indicating that the inelastic scattering that governs the temperature dependence is of the same origin and is from quantum critical fluctuations. A sub-linear temperature dependence is not anticipated in conventional models of criticality that only consider electron scattering from critical fluctuations of magnetization [4] . On the other hand, a similar sub- T linear behaviour in ρ has been reported in the unusual quantum critical metal YbRh 2 Si 2 (ref. 17 ), whose T 3/4 resistivity is interpreted in the context of a critical quasiparticle theory that includes the interaction of heavy quasiparticles with three-dimensional AFM fluctuations in the non-Gaussian critical region [18] . In this context for Sn-doped CeRhIn 5 , ρ c ( T ) should recover a normal metallic temperature-squared dependence at pressures higher than P c , which it does. As illustrated in Fig. 2d , ρ 0 decreases to 47.2 μΩ cm and A is 0.56 μΩ cm K −2 , which corresponds to a Sommerfeld coefficient of 236 mJ mol −1 K −2 . The anomalous temperature dependence of the resistivity and strong enhancement of ρ 0 and A at P c imply that the putative QCP lies at P c , the pressure where T c ( P ) is highest (see Fig. 3b and Supplementary Note 3 ). 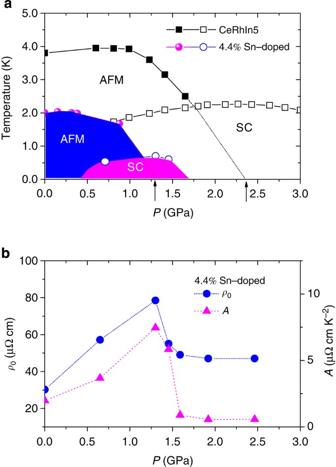Figure 3: Pinning ofTcmaximum via a QCP. (a) Resistively determined pressure–temperature phase diagrams are plotted at zero magnetic field for CeRhIn5(squares) and 4.4% Sn-doped CeRhIn5(circles). Solid symbols denote the antiferromagnetic (AFM) transition temperature (TN) and open symbols describe the superconducting transition temperature (Tc). The maximumTcis lower in Sn-doped CeRhIn5because of pair-breaking arising from strong impurity scattering. Arrows on thexaxis indicate the AFM QCPs at 1.3 GPa for 4.4% Sn-doped and at 2.3 GPa for pure CeRhIn5, respectively. (b) Pressure dependence of the residual resistivityρ0(circles) andT2coefficientA(triangles) ofρcfor 4.4% Sn-doped CeRhIn5are plotted on the left and right ordinates, respectively. These parameters were obtained by a least-squares fit of thecaxis electrical resistivity at 5 Tesla by usingρc=ρ0+AT2(seeSupplementary Note 4). Figure 3: Pinning of T c maximum via a QCP. ( a ) Resistively determined pressure–temperature phase diagrams are plotted at zero magnetic field for CeRhIn 5 (squares) and 4.4% Sn-doped CeRhIn 5 (circles). Solid symbols denote the antiferromagnetic (AFM) transition temperature ( T N ) and open symbols describe the superconducting transition temperature ( T c ). The maximum T c is lower in Sn-doped CeRhIn 5 because of pair-breaking arising from strong impurity scattering. Arrows on the x axis indicate the AFM QCPs at 1.3 GPa for 4.4% Sn-doped and at 2.3 GPa for pure CeRhIn 5 , respectively. ( b ) Pressure dependence of the residual resistivity ρ 0 (circles) and T 2 coefficient A (triangles) of ρ c for 4.4% Sn-doped CeRhIn 5 are plotted on the left and right ordinates, respectively. These parameters were obtained by a least-squares fit of the c axis electrical resistivity at 5 Tesla by using ρ c = ρ 0 + AT 2 (see Supplementary Note 4 ). Full size image Global temperature–pressure phase diagrams of pure CeRhIn 5 and 4.4% Sn-doped CeRhIn 5 are plotted in Fig. 3a . The similarity in the pressure dependence of the magnetic and SC phases of both compounds is apparent, although T N differs almost by a factor of two: (1) A pressure-induced dome of superconductivity exists in both systems, but the maximum T c is shifted from 2.3 GPa for the undoped to 1.3 GPa for the 4.4% Sn-doped CeRhIn 5 . (2) T N initially increases with increasing pressure, decreases with further pressure and abruptly disappears when the pressure-induced T c exceeds T N , suggesting that long-range AFM order arises from RKKY (Ruderman–Kittel–Kasuya–Yosida) interactions (see Supplementary Fig. 3 ). (3) A T c maximum occurs at the QCP for both compounds, confirming that critical quantum fluctuations are the source of unconventional superconductivity. (4) The dependence on temperature of ρ c at the QCP is sub-linear in the normal state, which reflects the unconventional nature of the QCP. Although there are many cases of superconductors near spin-density-wave QCPs [19] , [20] , [21] , [22] , [23] , [24] , superconductivity in a metal whose quantum criticality is unconventional [4] , for example, YbRh 2 Si 2 , CeCu 6− x Au x and CeRhIn 5 has been rare, raising a question whether the associated critical bosonic and fermionic fluctuations can provide the necessary attractive interaction to form Cooper pairs. Clear identification of the QCP in 4.4% Sn-doped CeRhIn 5 and its sub- T linear temperature dependence of ρ c in the normal state indicate that unconventional superconductivity is promoted by an unconventional QCP. Recent numerical calculations have found that singlet-pairing correlations are enhanced at such a QCP [25] . Nucleation of unconventional superconductivity at the respective QCPs of Sn-doped and pristine CeRhIn 5 attests that superconductivity is pinned to the QCPs because the associated critical fluctuations are the source of the pairing glue. These results provide a way to control unconventional superconductivity and motivate theoretical and experimental imperatives to elucidate the mechanism of QCP-induced superconductivity, especially in metals whose criticality involves both bosonic and fermionic degrees of freedom. Crystal synthesis and experiments in pressure Single crystals of CeRh(In 1− x Sn x ) 5 were synthesized by a standard In-flux technique. Basic physical properties of CeRh(In 1− x Sn x ) 5 were measured previously [12] . The c axis electrical resistivity measurements were performed under pressure for samples with a Sn concentration x =0.044, where the value of x was determined by microprobe analysis. Pressure work was performed using a hybrid Be–Cu/NiCrAl clamp-type pressure cell with silicone fluid as the pressure medium to ensure hydrostatic condition for pressure up to 2.5 GPa. Pressure in the cell was determined from the pressure-dependent SC transition temperature of a Pb manometer using the pressure scale of Eiling and Schilling [26] . A standard four-probe configuration, using spot-welded contacts, was used to measure the c axis electrical resistivity with an LR700 Resistance Bridge. Two different cryostats were used to control temperature and magnetic field: a 4 He cryostat for temperature measurements from 300 to 1.2 K and a 3 He cryostat for temperatures from 10 down to 0.3 K and for magnetic fields up to 5 Tesla. How to cite this article: Seo, S. et al . Controlling superconductivity by tunable quantum critical points. Nat. Commun. 6:6433 doi: 10.1038/ncomms7433 (2015).